Red blood cell as an adaptive optofluidic microlens The perspective of using live cells as lenses could open new revolutionary and intriguing scenarios in the future of biophotonics and biomedical sciences for endoscopic vision, local laser treatments via optical fibres and diagnostics. Here we show that a suspended red blood cell (RBC) behaves as an adaptive liquid-lens at microscale, thus demonstrating its imaging capability and tunable focal length. In fact, thanks to the intrinsic elastic properties, the RBC can swell up from disk volume of 90 fl up to a sphere reaching 150 fl, varying focal length from negative to positive values. These live optofluidic lenses can be fully controlled by triggering the liquid buffer’s chemistry. Real-time accurate measurement of tunable focus capability of RBCs is reported through dynamic wavefront characterization, showing agreement with numerical modelling. Moreover, in analogy to adaptive optics testing, blood diagnosis is demonstrated by screening abnormal cells through focal-spot analysis applied to an RBC ensemble as a microlens array. Red blood cell (RBCs) anomalies are significant symptoms for identification of health disorders. In particular, several blood diseases involve modification in the morphology of such cells, that is, sickle-cell disease, malaria and spherocytosis [1] , [2] , [3] . For these reasons, many non-invasive optical imaging systems have been developed for the investigation of RBC morphology as a diagnostic clinical factor [4] , [5] , [6] , [7] , [8] . In particular, quantitative phase-contrast methods have been explored for three-dimensional (3D) shape retrieving of live and unlabelled erythrocytes measuring volumes, refractive indexes and morphological parameters [9] , [10] , [11] , [12] . However, all the aforementioned imaging methods require interferometric analysis and/or complex image processing for morphology retrieval in two-dimensional and 3D and, most important, the diagnosis is subjective, as it depends on the physician’s personal evaluation of such images. Moreover, huge steps forward have been taken in the last years in the field of photonic techniques applied to medical science with the aim to make less invasive and more efficient current therapies or for developing new ones. In particular, challenging results have been obtained by enlarging the potential capabilities of optical tweezers (OTs) as a no-contact tool for cell manipulation [13] , [14] , [15] . Recently, for the first time, optical trapping has been aimed in vivo at manipulating RBCs within subdermal capillaries on living mice [16] . At the same time, many efforts have been spent to go towards the miniaturization of a photonic device that could open new ways for endoscopic analysis [17] , [18] , [19] . In this context, we propose a new concept where cells can be manipulated and adopted as functional and active optical elements. Specifically, we model RBCs as optofluidic nanomicrolenses [20] , [21] , [22] by demonstrating, in vitro , their focus tunability and imaging capability. Human erythrocytes, in their mature state and under physiological and healthy conditions, are flexible biconcave disks with homogeneous distribution of the refractive index. By an optical point of view, we will take benefit of the intrinsic great deformability [23] , [24] , [25] and the lack of nucleus and organelles [26] thus modelling and demonstrating that an RBC is a sort of disk-shaped microstructured envelope that changes its shape and is exploitable as a tunable liquid-lens. In fact RBCs are very flexible and their deformability allows them to bring oxygen even through the smallest capillaries in the vascular system. RBC morphology variation is achievable by triggering the liquid buffer osmolarity thus permitting swelling from the biconcave microfluid disk, with a volume of about 90 fl, up to a sphere reaching 150 fl. By considering the RBC average refractive index [4] ranging between 1.38 and 1.42 immersed in a liquid buffer with lower refractive index (1.334), we show that this focal length can change in a range of about 20 μm, from deep negative values to positive ones. A further functionality that we exploit here is about blood diagnostics. Here we demonstrate that, by exploiting the new concept of bio-microlenses and in analogy to indirect adaptive optics (IAO)-testing tools (that is, Shack–Hartmann) [27] , it is possible to discern between healthy and anomalous RBCs, thus providing a completely new, faster and much more objective diagnostic criterion. We will validate the RBC-focusing properties for providing full morphology identification. Any classical shape retrieval and conventional image-processing analysis will not be necessary. Examples of fast blood screening, 3D morphology retrieval and imaging properties of the RBC lens are reported. RBC focal length tunability RBC is modelled as a pure phase object, and simulation is performed implementing a modification of the formula for the ideal RBC biconcave shape [28] (see Supplementary Methods 1 and Supplementary Figs 1 and 2 for details). We consider a monochromatic plane wave propagating thorough it that behaves as an aberrated lens. Therefore the diffracted wavefront at the exit pupil of the microlens, computed using a phase-retrieval approach [29] , is expressed as a linear combination of Zernike polynomials [30] , [31] , [32] , [33] . Through computation we noted that the focal properties of normal discocyte are mainly due only to the first two quadratic polynomial terms, which correspond to the contributions of Zernike coefficients of order 4 and 12, that is, focus shift, a 4 , and third-order spherical aberrations, a 12 , while other terms are negligible. Meanwhile spherocytes (Methods) can be described essentially only by a focus-shift term, a 4 . To demonstrate the different focal properties between discocytes and spherocytes, we employ interference (that is, digital holography (DH)) microscopy (see Methods) [34] , [35] , [36] , [37] , [38] . Specifically, to prove the tunable focal length of an RBC optofluidic lens, we manage a dynamic experiment switching a single RBC between discocyte (mainly a negative lens) to spherocyte (a positive lens). Noteworthy, RBCs change shape in a reversible way by varying buffers’ osmolarity (see Methods). RBC sample, immersed in isotonic solution, is injected into a micro-channel. Soon after, a hypotonic solution is introduced causing, in about 10 s, significant RBC swelling. Variation of the erythrocyte shape and consequent focal-length shifts are monitored in real time using the holographic microscope. Despite a discocyte being quite a complex lens, its focal length changes in a very clear way. Essentially, in a more accurate model, it is a lens having a strong spherical aberration. While the inner part (that is, for paraxial rays) has a negative focal length, the edges behave as a sort of toroid lens having a positive focal length for no-paraxial rays. The induced swelling of the RBC causes the substantial change of its shape, thus cancelling the central concavity. Consequently, the virtual focus (that is, negative focal spot) disappears completely while a reinforcement of the real focal spot occurs The experimental results fully confirm this behaviour as shown in Fig. 1 and Supplementary Movie 1 , where real-time measurements are compared with theoretical expectations, thus showing noteworthy agreement. In Fig. 1a , the diffraction propagation of the retrieved complex wavefront along the optical axis is reported. Wavefront is retrieved by numerical reconstruction of a real-time digital holographic recording during the experiment. The intensity distributions, in the transverse plane and along the optical axis (plane x – z ), show very distinctly that, for a spherocyte RBC, the virtual focal spot vanishes completely, while the discocyte is swelling (see Supplementary Movie 1 ). Focal-length change during RBC swelling is also confirmed by a wavefront Zernike analysis reported in Fig. 1 and Supplementary Movie 2 , where Zernike shape fitting ( Fig. 1b ) and principal Zernike coefficients ( Fig. 1c ) are calculated. It should be noted that, the theoretical trends of Zernike coefficients (left of Fig. 1c ) show how the spherical aberration goes to zero; meanwhile focus shift is maximized. The same happens in the experimental case (right of Fig. 1c ), for which virtual and real focal lengths of an RBC, that is, before and after its swelling, can be directly derived by Zernike coefficients. In particular, the RBC in Fig. 1 presents in this case virtual foci before the sample plane at about −7.4 μm while its real focus, after hypotonic solution adding, is calculated at a distance of about 10.8 μm. Detailed model of discocyte RBC by Zernike polynomials is described in the Supplementary Methods 1 ; Supplementary Figs 1 and 2 . We report in Fig. 1d only the simulated maximum intensity peak correspondent to the virtual focus. The entire simulation results on the light intensities distribution is shown in Supplementary Movie 3 . In literature, the scattering theory [39] , [40] is considered for interaction of light with RBCs. However, the model described here is in the framework of geometrical optics and furnishes a good approximation of the interaction between light and the RBC lens. 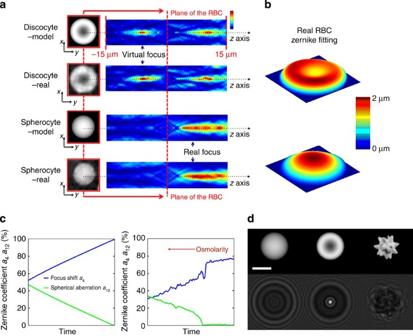Figure 1: RBC behaves as a microlens. (a) The left part presents the phase-shifts in plane (x–y) for a single RBC, simulated and real both discocyte and spherocyte. On the right, the correspondent light intensity distributions in the plane (x–z), for a plane monochromatic wave propagating from the left through the cell, are reported. RBC behaves as a tunable lens passing from a virtual focus to a real one by changing buffer osmolarity. Scanning range along thezaxis is between −15 and 15 μm.Supplementary Movie 1shows this process in real time. (b) The two retrieved wavefronts obtained from real RBC before and after swelling, whilecreports, both theoretically and experimentally, the energy percentage of Zernike coefficients, during the hypotonic solution addition (during swelling spherical aberration goes to zero, meanwhile focus shift is maximized).Supplementary Movie 2shows the Zernike-fitting outputs and the focusing coefficients variation in real time. (d) Simulation results: in the top row are three simulated RBC shapes; in the bottom row the maximum intensity occurs for discocyte in the plane (x–y) at a distancez=−7 μm from the RBC plane. Scale bar=5μm. Figure 1: RBC behaves as a microlens. ( a ) The left part presents the phase-shifts in plane ( x – y ) for a single RBC, simulated and real both discocyte and spherocyte. On the right, the correspondent light intensity distributions in the plane ( x – z ), for a plane monochromatic wave propagating from the left through the cell, are reported. RBC behaves as a tunable lens passing from a virtual focus to a real one by changing buffer osmolarity. Scanning range along the z axis is between −15 and 15 μm. Supplementary Movie 1 shows this process in real time. ( b ) The two retrieved wavefronts obtained from real RBC before and after swelling, while c reports, both theoretically and experimentally, the energy percentage of Zernike coefficients, during the hypotonic solution addition (during swelling spherical aberration goes to zero, meanwhile focus shift is maximized). Supplementary Movie 2 shows the Zernike-fitting outputs and the focusing coefficients variation in real time. ( d ) Simulation results: in the top row are three simulated RBC shapes; in the bottom row the maximum intensity occurs for discocyte in the plane ( x – y ) at a distance z =−7 μm from the RBC plane. Scale bar=5μm. Full size image RBC-biolens imaging properties We performed a simple experimental test to demonstrate the imaging capability of an RBC. A spherocyte RBC is used to image a sub-micrometre pattern achieving an increased magnification of about 20%. For demonstrating the magnifying properties of the biolens in hypotonic solution, we inserted a piece of a digital versatile disc (DVD) (780 nm pitch) between the light source and the RBC, behaving as a biconvex lens. By considering the distance between the RBC and the grating fixed at 16 μm, and by making the approximation that a spherocyte is a thin convergent lens, with focal length equal to 9 μm, we calculate a real image with magnification M th =1.29. In Fig. 2a a schematic view of the experiment is showed. In Fig. 2b,c a comparison between a portion of the DVD grating and the same magnified portion seen through the biolens is reported. We observe an increase in the mumber of pixels (from 26 to 32) in the magnified image of one grating period, which corresponds to M exp ≈1.22, quite in agreement with the calculated value. 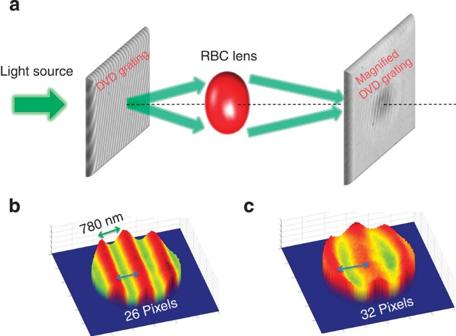Figure 2: RBC imaging properties. (a) Schematic view of the imaging test. A piece of a DVD is inserted as a test object between the light source and the RBC in hypotonic solution, the latter behaving as a biconvex lens. (b,c) Comparison between the grating and its magnified image thorough the biolens. Figure 2: RBC imaging properties. ( a ) Schematic view of the imaging test. A piece of a DVD is inserted as a test object between the light source and the RBC in hypotonic solution, the latter behaving as a biconvex lens. ( b , c ) Comparison between the grating and its magnified image thorough the biolens. Full size image Successively, we have used OTs (see Methods) to manage the position in 3D of the RBC. Magnified image of the DVD grating is visible in the centre of the cell. Supplementary Movie 4 describes the whole raster-scanning process while the RBC lens is moved first vertically along the optical axis, then in the transversal plane. The distortion of the magnified lines of the grating is due to the spherical aberration of the lens (see Fig. 2c ). These results demonstrate that RBC can behave as a tunable and optofluidic lens, having an imaging capability. Real-time blood screening through focal-spot aberrations Once it is proved that an RBC can be seen as an optofluidic microlens, it is possible to assert that any specific RBC morphology has its own focusing property. Since any blood disease has a typical shape, this implies that erythrocytes presenting more complicated shapes or deviations from normal healthy cases can be definitely identified by their focal spots, thus allowing blood disorder identification. In fact, any deviation from the healthy RBC morphology can be read as a sum of aberrations in the propagated optical wavefront passing through the cells, exactly as it occurs for any optical system. First, we analysed separately two different samples, made of hundreds of RBC, in two different osmolarity conditions. We performed numerous tests to get data from a statistical point of view, with the aim to estimate the focal-length ranges useful to determine the percentage of healthy cells in a crowded RBC ensemble. For the spherocyte ensemble, we measure real foci in front of the microlens array at a distance of about 9.72 μm while the discocyte ensemble presents virtual foci before the sample plane at about −6.33 μm. The corresponding s.d. are 1.06 and 0.84 μm. The results are displayed in Fig. 3a,b . Viewing the RBC ensemble as an array of microlenses is, in principle, a very powerful diagnostic tool. In fact, by exploiting all the base concepts of IAO, an RBC’s full 3D morphometry can be retrieved. The innovative diagnostic aspect is demonstrated in Figs 4 and 5 and Supplementary Movie 5 . The all-optical-based analysis is performed illuminating the sample with monochromatic light, necessary to have a definite focusing effect that otherwise cannot be obtained (chromatic aberrations hinder the formation of sharp focal spots as displayed in Fig. 3c ). It is important to note that no interferometry is required. A very fast pre-screening test is realized where the output establishes the percentage of healthy cells from the evaluation of the spot ellipticity in the virtual focus plane. Results are reported in Fig. 4 and Supplementary Movie 5 . Visualization of the spots and percentage of detected healthy and doubtful cells are furnished simultaneously, thanks to the test characteristic to be quasi real time. To validate the pre-screening process, we conducted a more sophisticated analysis based on the IAO [27] to have deeper information on the real cell shape. The optical intensities in the plane behind the RBCs are recorded for the entire field of view. For each intensity focal spot, an iterative Fourier transform algorithm calculate the wavefront aberrations where the output phase is modelled as a combination of Zernike polynomials making the assumption that only tilts, focus shift, spherical aberration, astigmatism and coma terms are present. Zernike coefficients for normal discocytes are essentially two, that is, focus shift and spherical aberration terms that justify the presence of the virtual focus in the plane before the RBC ensemble. Conversely, spherocytes present the focus coefficient several orders of magnitude higher than the others thus resulting in real foci. 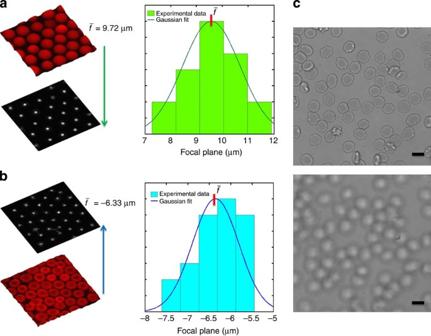Figure 3: Focusing of an RBC ensemble. (a,b) Static test: phase-contrast reconstructions in the image plane and intensity reconstructions in average focal planes of two samples of RBCs in different osmolarity conditions and investigation of corresponding focusing properties. In both cases, RBCs are analysed to retrieve their focal lengths from which average and s.d. values are calculated (see histograms on the right). (c)Typical white-light images of an RBC sample in focus and out of focus. No sharp focal spots can be detected. Scale bar, 5 μm (for both images). Figure 3: Focusing of an RBC ensemble. ( a , b ) Static test: phase-contrast reconstructions in the image plane and intensity reconstructions in average focal planes of two samples of RBCs in different osmolarity conditions and investigation of corresponding focusing properties. In both cases, RBCs are analysed to retrieve their focal lengths from which average and s.d. values are calculated (see histograms on the right). ( c )Typical white-light images of an RBC sample in focus and out of focus. No sharp focal spots can be detected. Scale bar, 5 μm (for both images). 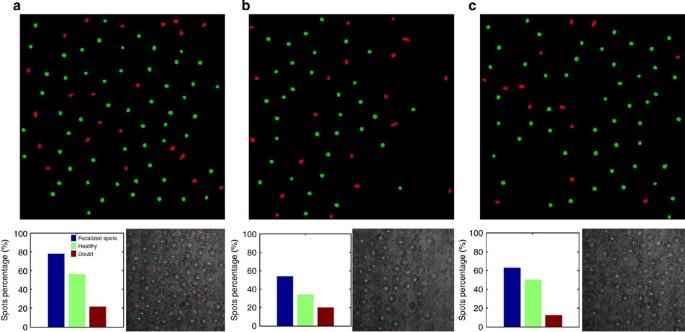Figure 4: RBC pre-screening process. (a–c) Frames ofSupplementary Movie 5where a real-time RBC’s pre-screening is performed, by analysing the intensity spots in the virtual focus plane (z=−6.33 μm). Healthy discocytes correspond to a quasi-circular intensity spot (green); red spots correspond to doubtful cases. The distinction between ‘healthy’ and ‘doubtful’ is obtained by evaluating the ratio between minor and major axes of a best-fit ellipse of each spot (ellipticity). The healthiness level is considered >0.8. Blue histograms represent the number of RBCs detected, green and red ones are the percentage of healthy and doubtful cases, respectively. For each of the three frames, the correspondent intensity images are reported to validate the unambiguous relation between spots and cells. Full size image Figure 4: RBC pre-screening process. ( a – c ) Frames of Supplementary Movie 5 where a real-time RBC’s pre-screening is performed, by analysing the intensity spots in the virtual focus plane ( z =−6.33 μm). Healthy discocytes correspond to a quasi-circular intensity spot (green); red spots correspond to doubtful cases. The distinction between ‘healthy’ and ‘doubtful’ is obtained by evaluating the ratio between minor and major axes of a best-fit ellipse of each spot (ellipticity). The healthiness level is considered >0.8. Blue histograms represent the number of RBCs detected, green and red ones are the percentage of healthy and doubtful cases, respectively. For each of the three frames, the correspondent intensity images are reported to validate the unambiguous relation between spots and cells. 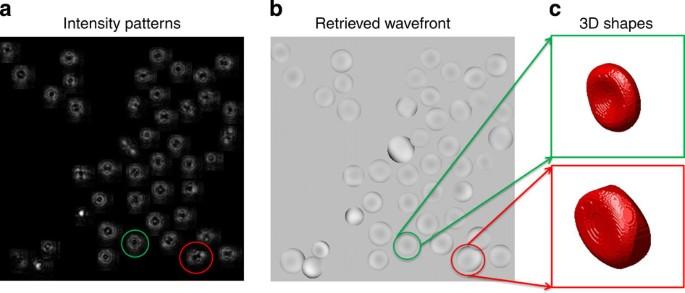Figure 5: RBCs shape retrieval from spot analysis. (a) Intensity patterns at the real focus plane. (b) For each spot, the corresponding wavefront is calculated to retrieve the phase distribution able to generate such intensity spots, which is computed by a combination of Zernike polynomials for each retrieved. The results for all the spots of the ensemble are displayed. (c) 3D morphology of two RBCs are shown. Full size image Figure 5: RBCs shape retrieval from spot analysis. ( a ) Intensity patterns at the real focus plane. ( b ) For each spot, the corresponding wavefront is calculated to retrieve the phase distribution able to generate such intensity spots, which is computed by a combination of Zernike polynomials for each retrieved. The results for all the spots of the ensemble are displayed. ( c ) 3D morphology of two RBCs are shown. Full size image Finally, abnormal shapes present the other coefficients with non-negligible values. Interestingly, the retrieved wavefront expressed by the Zernike polynomials can be used for full 3D morphological visualization under symmetry assumptions [41] (see Fig. 5c ). The approach presented can be applied to samples made of hundreds of cells supplying information on each RBC present in the ensemble as shown in Fig. 5 . Detailed description of RBC shape retrieval is reported in the Supplementary Methods and Supplementary Figs 3 and 4 . The approach can be proposed as an optics-based diagnostic tool. In fact, RBC focus-footprint is a clear and simple marker about its morphology for a fast easy pre-screening in vitro analysis. In fact, as shown in Fig. 4 , the method is able to detect easily the percentage of normal discocytes in an ensemble by evaluating the number of spots and their ellipticity in the calculated virtual focal plane ( z =−6.33). In case the percentage of discocytes (that is, healthy cells) is low with respect to an a-priori fixed value, further and deeper analysis can be considered for retrieving abnormal RBC shapes by processing the spots’ intensities in the calculated real focal plane ( z =9.72), as demonstrated in the results of Fig. 5 . In this paper, RBCs are modelled as optofluidic microlenses with well-defined optical properties. Experimental evidences, numerical simulations and final practical application have been provided for this new concept. From the tunability experiment reported in Fig. 1 and the experimental results in Fig. 3 , it is clear that spherocyte and discocyte have opposite concavities, therefore they focus laser light at real and virtual foci, behind and before the lens, respectively, thus confirming that an RBC can be considered as an optofluidic lens able to change its focal length from negative to positive values. In ref. 42 , the physical properties (refractive index, shape and volume) of RBCs are characterized for several buffer’s osmolarities. We demonstrated here that the focal length depends also on the buffer chemistry and it is strictly related to such physical parameters. Therefore, in the tuning experiment, by defining the medium osmolarity, we control the final stage of RBCs in terms of focal lengths. We demonstrated the magnifying properties of the RBC when it is employed as an active lens. Indeed, a grating with a pitch of 780 nm is imaged through the RBC lens resulting in a magnification of about 1.22. Moreover, by using OTs, the RBC lens is moved in three dimensions to ‘scan’ a little part of the grating, thus behaving as a ‘guided magnifying lens’ that can be foreseen as a sort of raster-scanning imaging inside the human body. Finally, a new paradigm is opened on biomedical application. In fact, by seeing RBCs as microlens array, there is the possibility to discriminate normal healthy cells from all other abnormal shapes by analysing optical focal spots with a monochromatic or quasi-monochromatic light source. We discuss and show that the method is fast and effective and allows for unambiguous identification of discocytes RBC from all the abnormal ones by evaluating the spots ellipticity in the virtual focus plane. Such a pre-screening procedure is based on the fact that normal discocyte biolenses present focus spots placed along the optical axis but in the opposite direction with respect to the abnormal ones. Furthermore, we prove that 3D RBC shape can be evaluated through the analysis of focal spots in the biolens forward focal plane. The presented approach is developed in analogy to wavefront aberration analysis by IAO, a well-known technology usually employed in astronomy as well as in optical communications and sensing. We demonstrate that focal spots are strictly correlated to the morphology as shown in Fig. 5 . Consequently, future blood diagnosis can be achieved by abandoning the concept of diagnosis through classical imaging. The concept demonstrated here is disruptively new. In fact, at the best of our knowledge, it is the first time that a cell can be assumed as an active and tuneable lens. Experimental evidence of tunability, imaging and diagnostics reported here demonstrate in full the in vitro proof of principle. In our opinion, this could open the route for potential impacts either for future blood diagnostics and in vivo endoscopy. Recent improvement in biophotonics as the manipulation of RBCs from the outside of the vein [16] and, at the same time, new papers on the miniaturization of OT on a single fibre [17] , [43] , [44] could convincingly lead to envisage an integration of the presented technique for endoscopy. For example, it could be investigated a fibre-based system able to manipulate and trap RBCs inside the vein. The application could be the imaging of the RBC themselves to perform diagnosis. Indeed, by the same authors, the possibility to image a fixed object hidden by a dense flow of RBCs has been recently proved [45] . In particular in the Fig. 4d of such paper fixed RBCs are clearly visible thorough a dense layer of flowing erythrocytes. Concerning in vitro blood screening, the important improvement of the presented technique is that neither image segmentation nor traditional phase computing is required, thus resulting in quasi real-time output. In fact, as shown in Fig. 5 , the analysis just needs the map of the focal spots to accomplish pre-screening. Thus the proposed technique could be able to easily detect blood disorders involving shape abnormalities, for example, sickle-cell disease, spherocytosis, elliptocytosis and malaria. Moreover, it is expected that the device for such a diagnostic tool could be adapted at lab-on-chip scale, because the optical set-up is very easy as it uses only a camera and a laser light source in the visible range that indeed nowadays are very compact and of low cost. Sample preparation and isolation of erythrocytes All experiments were done with heparinized blood drawn within the hour before use. Healthy blood was collected from one of the co-authors, who gave informed consent. The sample was prepared as follows: ~3 ml of heparinized whole blood was withdrawn into a haematocrit tube. Blood was centrifuged at room temperature, for 15 min at 2,500 r.p.m. to separate it into its component parts (plasma, buffy coat and RBCs at the bottom of the centrifuge tube). The pellet (≈1.5 ml) was collected and 100 μl of erythrocytes were diluted with a saline solution of 0.90% w/v of sodium chloride (NaCl) in sterile water up to a final volume of 2 ml. The osmolarity of the medium was about 308 mOsm l −1 and it was isotonic with the membrane of RBCs. No visible haemolysis occurred. For the hypotonic and hypertonic solutions, we used a medium osmolarity of about 205 and 410 mOsm l −1 , respectively. When RBCs are in a hypotonic environment, the cell interiors accumulate water that flows across the cell membrane into the cell, causing it to expand. On the contrary, when the environment is hypertonic, the cell eliminates water and shrinks. Finally, in an isotonic solution, water exchange between the cell and the environment is balanced, and no change in cell volume occurs. These situations are described in Supplementary Fig. 1 , resulting in different shapes of the cells depending on the tonicity of the solution. Digital holography and the OT apparatus We integrate a microscope based on DH arrangement and an OT modulus to simultaneously image and manipulate biological samples [31] , [34] ( Fig. 6 ). The DH set-up is made by a 400 -mW at 532 nm fibre-coupled laser that acts as a source for a Mach–Zehnder interferometer ( Fig. 6 ), whose main beam is directed into a customized inverted microscope equipped with an oil immersion × 100 microscope objective, allowing bright-field imaging of the cells. The reference beam is recombined with the first one by a beam splitter generating interference fringe patterns (called digital holograms) of the samples that are recorded by a 1,024 × 1,024 charge-coupled device camera (AVT Technologies). The OT apparatus is realized by using a 3-W infrared laser source in combination with a Phase Only Spatial Light Modulator (by Holo-Eye), with the aim of trapping and moving multiple RBC lenses in 3D. In particular, the OT modulus is used to demonstrate the imaging properties of RBCs ( Supplementary Movie 4 ). The trapping laser emits at 1,064 nm; the beam is expanded to fit the aperture of the spatial light modulator operating in reflection mode. Then, the laser beam is injected into the microscope objective (mumerical apperture=1.25) thorough a standard 4f optical configuration (not shown for simplicity). RBCs (after separation from the other blood cells) are placed in a Petri dish and analysed by this apparatus. 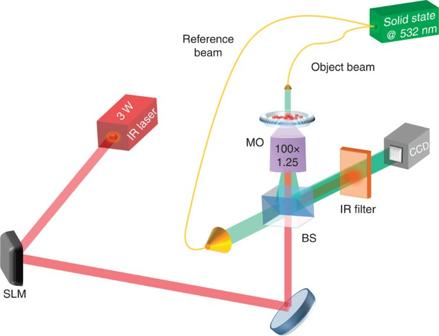Figure 6: Optical experimental arrangement. DH-OT set-up for simultaneous imaging and trapping. DH set-up is based on a Mach–Zehder interferometer where the object beam passes through the sample and then it is led to interfere with the reference beam by a Beam Splitter cube (BS). The interferograms are recorded by the camera (charge-coupled device (CCD)). The OT arrangement is realized by an infrared (IR) laser emitting at 1,064 nm. Multiple traps are managed by the spatial light modulator (SLM) inserted into the set-up following the standard 4f configuration. A filter is used to avoid the IR laser intensities that could be recorded during the experiments. Both DH and OT lasers paths are aligned in a 100x high-numerical aperture microscope objective (MO). Figure 6: Optical experimental arrangement. DH-OT set-up for simultaneous imaging and trapping. DH set-up is based on a Mach–Zehder interferometer where the object beam passes through the sample and then it is led to interfere with the reference beam by a Beam Splitter cube (BS). The interferograms are recorded by the camera (charge-coupled device (CCD)). The OT arrangement is realized by an infrared (IR) laser emitting at 1,064 nm. Multiple traps are managed by the spatial light modulator (SLM) inserted into the set-up following the standard 4f configuration. A filter is used to avoid the IR laser intensities that could be recorded during the experiments. Both DH and OT lasers paths are aligned in a 100x high-numerical aperture microscope objective (MO). Full size image How to cite this article: Miccio, L. et al . Red blood cell as an adaptive optofluidic microlens. Nat. Commun . 6:6502 doi: 10.1038/ncomms7502 (2015).